Structural analyses of the chromatin remodelling enzymes INO80-C and SWR-C INO80-C and SWR-C are conserved members of a subfamily of ATP-dependent chromatin remodelling enzymes that function in transcription and genome-maintenance pathways. A crucial role for these enzymes is to control chromosomal distribution of the H2A.Z histone variant. Here we use electron microscopy (EM) and two-dimensional class averaging to demonstrate that these remodelling enzymes have similar overall architectures. Each enzyme is characterized by a dynamic ‘tail’ domain and a compact ‘head’ that contains Rvb1/Rvb2 subunits organized as hexameric rings. EM class averages and mass spectrometry support the existence of single heterohexameric rings in both SWR-C and INO80-C. EM studies define the position of the Arp8/Arp4/Act1 module within INO80-C, and we find that this module enhances nucleosome-binding affinity but is largely dispensable for remodelling activities. In contrast, the Ies6/Arp5 module is essential for INO80-C remodelling, and furthermore this module controls conformational changes that may couple nucleosome binding to remodelling. ATP-dependent chromatin remodelling enzymes use the energy from ATP hydrolysis to disrupt histone–DNA interactions, catalysing the ‘sliding’ of histone octamers in cis along with DNA, eviction of histone H2A/H2B dimers or ejection of an entire histone octamer [1] . A subset of these enzymes can also remove one or both histone H2A/H2B dimers from a nucleosome and replace it with a different H2A/H2B dimer, a reaction termed dimer exchange. Chromatin remodelling enzymes were initially identified as transcriptional regulators, but it is now clear that these enzymes impact nearly all nuclear processes [1] . Each remodelling enzyme harbours a catalytic ATPase subunit that is related to the ancient SF2 superfamily of DNA-dependent ATPases, and biochemical studies have defined four families of enzymes—SWI/SNF, ISWI, Chd1/Mi-2 and INO80, named after their founding members. Yeast INO80-C and SWR-C are two well-characterized members of the INO80 family of remodelling enzymes, and they are unique from other enzymes in that they catalyse the ATP-dependent exchange of histones from nucleosomal substrates [2] . Whereas SWR-C catalyses the ATP-dependent eviction of nucleosomal H2A/H2B and replaces them with H2A.Z/H2B variant dimers [3] , INO80-C promotes the opposite dimer exchange reaction [4] . Consequently, cells that lack SWR-C have very low levels of the histone H2A.Z variant within chromatin [3] , [5] , [6] , whereas inactivation of INO80-C leads to an aberrant pattern of H2A.Z distribution [4] . In addition to its dimer exchange activity, INO80-C is also able to perform more typical remodelling reactions, such as mobilizing nucleosomes in cis and influencing nucleosome spacing [7] . In contrast, SWR-C is inactive in all other types of remodelling assays, and thus appears to be dedicated to H2A.Z deposition [4] . Both INO80-C and SWR-C are large (>1 MDa), multi-subunit assemblies that harbour related ATPase subunits, Ino80 and Swr1, respectively. These enzymes also share four subunits—Rvb1, Rvb2, Arp4 and Act1 (actin). The Rvb1 and Rvb2 subunits are highly related AAA + ATPases that bind to the central ATPase domains of Ino80 and Swr1, whereas the common Arp4 and Act1 subunits interact with the conserved HSA domain, positioned N-terminal to the Swr1 or Ino80 ATPase domains [8] , [9] , [10] . INO80-C and SWR-C complexes also harbour nine to ten complex-specific subunits. For INO80-C, the Arp8 subunit forms a subunit module with the Arp4 and Act1 subunits (Arp8/Arp4/Act1), and previous studies have suggested that this module is key for remodelling activity and that it interacts with DNA and histones [10] , [11] . Likewise, SWR-C contains a group of complex-specific subunits, including Yaf9 and Bdf1, which interact with Arp4 and Act1 at the N-terminal Swr1 HSA domain [9] . Subunits within this module are important for catalysis of H2A.Z deposition [9] . In addition, both INO80-C and SWR-C contain complex-specific modules that interact with Rvb1/Rvb2 within the ATPase domain–the Ies6/Arp5 subunit module within INO80-C appears to be essential for remodelling activities of INO80-C, and the Swc2/Swc3/Swc6/Arp6 module within SWR-C appears to govern the substrate specificity of the dimer exchange reaction [9] , [12] . Thus, the ATPase subunits for both INO80-C and SWR-C function as catalytic scaffolds that assemble subunit modules that regulate remodelling activity. Structural studies of chromatin remodelling enzymes have provided important insights into nucleosome recognition and remodelling mechanism. For instance, high-resolution crystal structures of the monomeric Chd1 and ISWI enzymes have led to models for how histone N-terminal domains and DNA might regulate their remodelling reactions [13] , [14] , [15] . Electron microscopy (EM) maps of the related SWI/SNF and RSC remodelling enzymes have revealed that these ∼ 1-MDa complexes interact with their nucleosomal substrates within either a shallow cleft on the enzyme surface or a large protein-ringed cavity [16] , [17] , [18] , [19] . In the case of INO80 complexes, high-resolution structures are available for the actin-related proteins, Arp8 and Arp4 (refs 20 , 21 , 22 ). Recently, two groups have presented EM reconstructions of the yeast INO80-C and SWR-C remodelling enzymes [11] , [23] . Interestingly, despite the large degree of functional and structural homology between the two complexes, these two structural studies presented quite different architectures. In the case of INO80-C, the data suggested an elongated structure, punctuated by a dodecameric Rvb1/Rvb2 ring at one terminus and the Arp8/Arp4/Act1 module at the other. In contrast, the SWR-C structure indicates a highly compact structure, with a single heterohexameric Rvb1/Rvb2 ring. Here we employ EM and two-dimensional (2D) class averaging to identify and directly compare the structures of yeast INO80-C and SWR-C. We find that both enzymes are quite variable in structure, but show remarkably similar overall features. Both enzymes have a population of elongated molecules that is exemplified by a flexible ‘tail’ domain and a globular ‘head’. Each of the head domains is composed of ring-like structures with sixfold symmetry, and mass spectrometry analyses of subunit stoichiometry indicate that each head is composed of a single heterohexameric Rvb1/Rvb2 ring. In addition to these elongated complexes, both INO80-C and SWR-C exhibit compact forms in which the tail domain appears to interact with the head. Analysis of INO80-C that lacks the Arp8/Arp4/Act1 module places these subunits within the tail domain. We find that this module is not essential for INO80-C ATPase or remodelling activities, but rather the Arp8/Arp4/Act1 module enhances nucleosome-binding affinity. In contrast, removal of the Ies6/Arp5 module inactivates all INO80-C activity and leads to an INO80-C that appears intact, but assumes a greater propensity to form the compact conformation. Likewise, removal of the related Swc2 module from SWR-C also appears to lead to a more compact state. Our results indicate that members of the INO80 family of chromatin remodelling enzymes are flexible assemblies capable of large-scale, regulated conformational changes that modulate nucleosome binding and enzymatic activity. EM of SWR-C and INO80-C reveal similar architectures INO80-C and SWR-C were purified to near homogeneity by tandem affinity purification from Ino80-TAP and Swr1-TAP yeast strains, respectively. SDS–polyacrylamide gel electrophoresis (PAGE) and mass spectrometry analyses confirmed the presence of the expected 15 INO80-C and 14 SWR-C subunits ( Supplementary Fig. 1 and Supplementary Tables 1 and 2 ; ref. 24 ). Samples were mildly cross-linked in preparation for EM analysis by adding glutaraldehyde directly to the final column elution. EM imaging of negatively stained INO80-C and SWR-C revealed a large degree of structural heterogeneity for both enzymes ( Fig. 1 ), with each enzyme population containing extended and compact forms (see also Supplementary Fig. 2 ). In contrast, parallel analysis of the yeast SWI/SNF complex yielded a more mono-disperse population that had features consistent with previous studies [17] . 2D class averages were calculated for both INO80-C and SWR-C, and the results indicated that the extended forms of both enzymes were composed of a long ‘tail’ domain, punctuated by a compact ‘head’ ( Fig. 1 and Supplementary Fig. 2 ). Furthermore, INO80-C contained an excess of extended forms (53% extended and 28% compact; the remaining particles could not be assigned), whereas SWR-C had a greater propensity to form a compact structure (22% extended and 54% compact; Fig. 1 and Supplementary Fig. 2 ). Notably, the tail domains for both enzymes appeared to be highly flexible, leading to a continuum of extended conformations. The head domain in both complexes has a diameter of about 13 nm, but the tail in the most extended INO80-C molecules appears to be somewhat longer, 23.4 nm, than in the most extended SWR-C molecules, 17.2 nm. 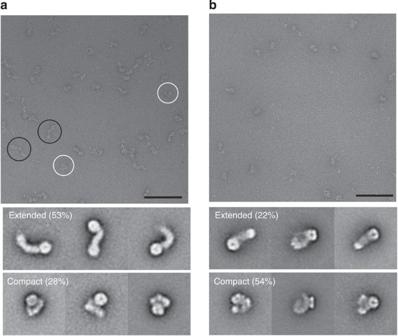Figure 1: EM analysis of yeast INO80-C and SWR-C. (a) Upper panel: EM image of negatively stained INO80-C, showing particles in extended (black circles) and compact (white circles) conformations. Scale bar, 100 nm. Lower panels: Selected class averages of INO80-C showing the complex in extended (upper panels) and compact conformations (lower panels). The numbers are percentages of each conformation in the entire population (10,128 particles; seeSupplementary Fig. 2for all averages). Side length of individual panels is 57.3 nm. (b) Upper panel: EM image of negatively stained SWR-C. Scale bar, 100 nm. Lower panels: Selected class averages of SWR-C showing the complex in extended (upper panels) and compact conformations (lower panels). The numbers are percentages of each conformation in the entire population (20,412 particles; seeSupplementary Fig. 2for all averages). Side length of individual panels is 57.3 nm. Figure 1: EM analysis of yeast INO80-C and SWR-C. ( a ) Upper panel: EM image of negatively stained INO80-C, showing particles in extended (black circles) and compact (white circles) conformations. Scale bar, 100 nm. Lower panels: Selected class averages of INO80-C showing the complex in extended (upper panels) and compact conformations (lower panels). The numbers are percentages of each conformation in the entire population (10,128 particles; see Supplementary Fig. 2 for all averages). Side length of individual panels is 57.3 nm. ( b ) Upper panel: EM image of negatively stained SWR-C. Scale bar, 100 nm. Lower panels: Selected class averages of SWR-C showing the complex in extended (upper panels) and compact conformations (lower panels). The numbers are percentages of each conformation in the entire population (20,412 particles; see Supplementary Fig. 2 for all averages). Side length of individual panels is 57.3 nm. Full size image Several 2D class averages revealed that the head domains of both INO80-C and SWR-C contain a ring structure with sixfold symmetry, reminiscent of the structure of Rvb1/Rvb2 hexameric rings [25] ( Fig. 2a,b ). Side views of the INO80-C and SWR-C head domains suggest that there may be two stacks of ring-like structures, although this is less distinct for SWR-C ( Fig. 2a,b ). 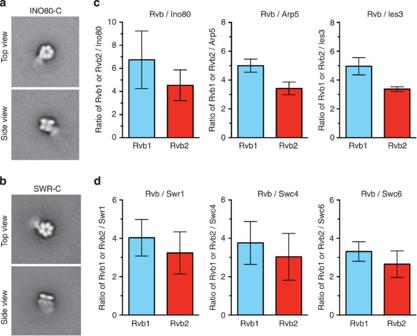Figure 2: INO80-C and SWR-C contain single hexameric rings of Rvb1/Rvb2. (a) Selected class averages of the head domain of INO80-C. Top view (top panel) shows a hexameric ring structure of Rvb1/Rvb2 (no symmetry was applied). Side view (bottom panel) depicts two layers of density. (b) Selected class averages of the head domain of SWR-C. Top view (top panel) shows a hexameric ring structure of Rvb1/Rvb2 (no symmetry was applied). Side view (bottom panel) depicts two layers of density. Side length of individual panels inaandbis 57.3 nm. (c,d) Rvb1 and Rvb2 subunit stoichiometries determined from mass spectrometry analyses for INO80-C (c) and SWR-C (d). Each error bar represents the standard deviation from three independent preparations. Figure 2: INO80-C and SWR-C contain single hexameric rings of Rvb1/Rvb2. ( a ) Selected class averages of the head domain of INO80-C. Top view (top panel) shows a hexameric ring structure of Rvb1/Rvb2 (no symmetry was applied). Side view (bottom panel) depicts two layers of density. ( b ) Selected class averages of the head domain of SWR-C. Top view (top panel) shows a hexameric ring structure of Rvb1/Rvb2 (no symmetry was applied). Side view (bottom panel) depicts two layers of density. Side length of individual panels in a and b is 57.3 nm. ( c , d ) Rvb1 and Rvb2 subunit stoichiometries determined from mass spectrometry analyses for INO80-C ( c ) and SWR-C ( d ). Each error bar represents the standard deviation from three independent preparations. Full size image To ensure that the different averages indeed represent different conformations of the complexes and not just different views, three-dimensional (3D) reconstructions were calculated using 60°/0° image tilt pairs. The particles selected from the images of the untilted specimens were classified into 100 or 150 groups. As previously observed, many of the INO80-C class averages showed extended particles, whereas the SWR-C class averages were dominated by more compact structures ( Supplementary Figs 3 and 4 ). Classes that produced similar averages were pooled (marked by asterisks in Supplementary Figs 3 and 4 ), and 3D reconstructions were calculated with the particle images from the tilted specimens ( Supplementary Fig. 5 ). Both maps reveal head and tail features, but with the tail in the INO80-C map adopting an extended conformation ( Supplementary Fig. 5a ) and that in the SWR-C map adopting a more bent conformation ( Supplementary Fig. 5b ). Despite their low resolutions ( ∼ 30 Å), the 3D maps confirm that the tails can adopt different conformations. INO80-C and SWR-C harbour single Rvb1/2 heterohexameric rings To obtain an accurate measurement of subunit stoichiometries within both INO80-C and SWR-C, three independent preparations of INO80-C and SWR-C were subjected to mass spectrometry analysis, and label-free spectral counting was used to provide a relative, quantitative measurement of subunit abundance ( Supplementary Fig. 1 and Supplementary Tables 1 and 2 ). Spectral counts were normalized to subunit length, and values for the Rvb1 and Rvb2 subunits were initially compared with either the Ino80 or the Swr1 subunits as they are predicted to be present at one copy per complex ( Fig. 2c,d ; ref. 17 ). Subsequently, two additional subunits from each complex were included in the analysis, as these subunits were consistently present at apparent equal stoichiometry with the ATPase subunit ( Fig. 2c,d , see also Supplementary Tables 1 and 2 ). In the case of SWR-C, the data are consistent with a single heterohexameric ring, as there was an average of 6.7 Rvb1/Rvb2 subunits per complex ( Fig. 2d and Supplementary Table 2 ). For INO80-C, the ratios of Rvb1 and Rvb2 subunits were slightly higher than those observed for SWR-C, with an average of 9.3 Rvb1/Rvb2 subunits per INO80-C complex ( Fig. 2c and Supplementary Table 1 ). These data are most consistent with both complexes containing a single heterohexameric ring, but the data suggest that INO80-C may contain additional copies of Rvb1/2 subunits. Structural and functional analysis of the Arp8 module To define the location of subunit modules that interact with the N-terminal domains of the ATPase subunits, INO80-C was purified from an arp8Δ strain. The resulting complex lacks the entire Arp8/Arp4/Act1 module that interacts with the Ino80 HSA domain ( Fig. 3a ). Samples were prepared for EM imaging, and 2D class averages demonstrated a loss of at least half of the tail domain, indicating that this module is located distal to the Rvb1/Rvb2 ring ( Fig. 3b and Supplementary Fig. 6 ), consistent with a recent study [11] . 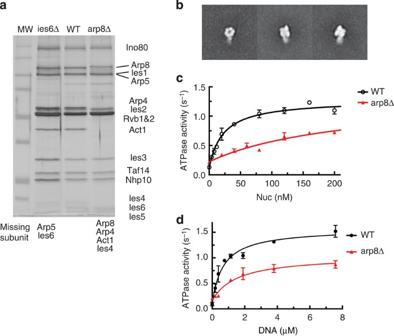Figure 3: Functional analysis of the INO80-Carp8subcomplex. (a) SDS–PAGE gel of INO80-C, INO80-Carp8and INO80-Cies6subcomplexes. (b) Selected class averages of negatively stained INO80-Carp8subcomplex. Top view (left panel) and side view (middle and right panels). Side length of individual panels is 57.3 nm. (c) Nucleosome-stimulated ATPase activity of the INO80-Carp8subcomplex. (d) DNA-stimulated ATPase activity of the INO80-Carp8subcomplex. Each error bar represents the standard deviation from three independent experiments. WT, wild type. Figure 3: Functional analysis of the INO80-C arp8 subcomplex. ( a ) SDS–PAGE gel of INO80-C, INO80-C arp8 and INO80-C ies6 subcomplexes. ( b ) Selected class averages of negatively stained INO80-C arp8 subcomplex. Top view (left panel) and side view (middle and right panels). Side length of individual panels is 57.3 nm. ( c ) Nucleosome-stimulated ATPase activity of the INO80-C arp8 subcomplex. ( d ) DNA-stimulated ATPase activity of the INO80-C arp8 subcomplex. Each error bar represents the standard deviation from three independent experiments. WT, wild type. Full size image Early studies of an INO80-C that lacked Arp8 suggested that this module is essential for both the ATPase and remodelling activities of INO80-C [10] . We re-evaluated the role of the Arp8/Arp4/Act1 module by performing detailed kinetic analyses of ATPase and remodelling activities. Analysis of the ATPase activity of wild-type INO80-C demonstrated that nucleosomes are a preferred substrate, as the K m for nucleosomes was at least tenfold lower than that for DNA ( Fig. 3c,d and Table 1 ). The INO80-C arp8 subcomplex exhibited a wild-type k cat for ATP hydrolysis, but the K m for nucleosomes increased approximately tenfold, and the K m for DNA increased approximately threefold ( Fig. 3c and Table 1 ). Surprisingly, this reduced affinity for nucleosomes as assayed by ATPase activity was not apparent when nucleosome binding of the INO80-C arp8 subcomplex was assayed by gel shift ( Fig. 4d ), suggesting that ATPase activity requires a distinct mode of nucleosome interaction. Table 1 ATPase parameters of INO80 complexes. 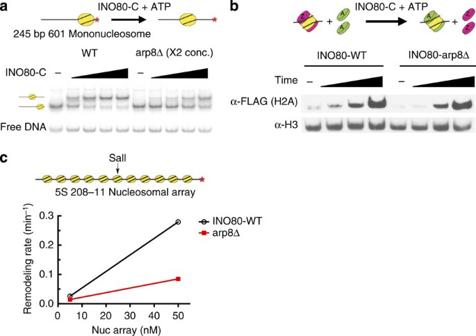Figure 4: The INO80-Carp8subcomplex is active for nucleosome remodelling. (a) Mononucleosome-sliding activity of the INO80-Carp8subcomplex. End-positioned mononucleosomes were incubated with twofold serial dilutions of INO80-C or INO80-Carp8(twofold higher concentration than wild type (WT)), and reactions were analysed by Native-PAGE. (b) Remodelling activity of the INO80-Carp8subcomplex on an 11-mer nucleosomal array substrate. Remodelling rates (min−1) are measured at 5 or 50 nM array concentration. (c) Dimer-exchange activity of the INO80-Carp8subcomplex. 5 nM INO80-C or INO80-Carp8were incubated with 100 nM H2A.Z mononucleosomes and 50 nM FLAG-tagged H2A/H2B dimers for 30, 60 or 120 min in the presence of 2 mM ATP. Reactions were analysed by Native-PAGE, and H2A incorporation was monitored by western blot analysis. Full size table Figure 4: The INO80-C arp8 subcomplex is active for nucleosome remodelling. ( a ) Mononucleosome-sliding activity of the INO80-C arp8 subcomplex. End-positioned mononucleosomes were incubated with twofold serial dilutions of INO80-C or INO80-C arp8 (twofold higher concentration than wild type (WT)), and reactions were analysed by Native-PAGE. ( b ) Remodelling activity of the INO80-C arp8 subcomplex on an 11-mer nucleosomal array substrate. Remodelling rates (min −1 ) are measured at 5 or 50 nM array concentration. ( c ) Dimer-exchange activity of the INO80-C arp8 subcomplex. 5 nM INO80-C or INO80-C arp8 were incubated with 100 nM H2A.Z mononucleosomes and 50 nM FLAG-tagged H2A/H2B dimers for 30, 60 or 120 min in the presence of 2 mM ATP. Reactions were analysed by Native-PAGE, and H2A incorporation was monitored by western blot analysis. Full size image Nucleosome remodelling activities for INO80-C and INO80-C arp8 were monitored in three separate assays. First, the ATP-dependent sliding of an end-positioned mononucleosome to a more central position was assayed in a native gel assay ( Fig. 4a ). The INO80-C arp8 subcomplex was partially active for nucleosome sliding, retaining ∼ 13% of wild-type activity. We then tested remodelling of a nucleosomal array substrate using a restriction enzyme-coupled reaction in which a unique SalI cleavage site is located within the central nucleosome of an 11-mer array [26] ( Fig. 4b ). Compared with wild-type INO80-C, the INO80-C arp8 subcomplex showed ∼ 50% activity at 5 nM array concentration and ∼ 30% activity at higher array concentrations ( Fig. 4b ). Finally, the role of the Arp8/Arp4/Act1 module in histone H2A/H2B dimer exchange was monitored using a mononucleosome-based assay [4] ( Fig. 4c ). In this assay, INO80-C catalyses the replacement of nucleosomal H2A.Z/H2B dimers with H2A/H2B dimers. Interestingly, INO80-C arp8 retained high levels of exchange activity ( Fig. 4c ). Similar results for all assays were obtained for two independent enzyme preparations. Thus, the Arp8/Arp4/Act1 module contributes to remodelling activities, most likely by enhancing nucleosome-binding affinity. The Ies6/Arp5 module is essential for INO80-C activities To identify the location and function of subunit modules that are associated with the ATPase domain, INO80-C was purified from an ies6Δ strain, and SWR-C was purified from an swc2Δ strain. The resulting INO80-C ies6 subcomplex lacked both Ies6 and Arp5 ( Fig. 3a ), and the SWR-C swc2 subcomplex was depleted for Swc2, Swc3, Swc6 and Arp6 (ref. 24 ). EM imaging of these subcomplexes failed to reveal a loss of protein density, likely due to the small size of these modules and their predicted location directly adjacent to the Rvb1/Rvb2 head domain ( Fig. 5a and Supplementary Figs 7 and 8 ). Interestingly, loss of either the Ies6 or the Swc2 module decreased the proportion of extended complexes and led to a higher percentage of compact forms for both INO80-C and SWR-C ( Fig. 5a ). 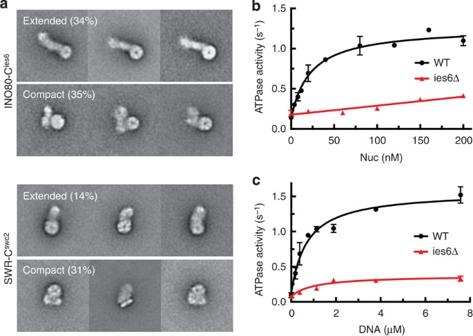Figure 5: Structural and functional analysis of INO80-Cies6and SWR-Cswc2subcomplexes. (a) Selected class averages of negatively stained INO80-Cies6and SWR-Cswc2subcomplexes showing extended (upper panels) and compact conformations (lower panels). The numbers are percentages of each conformation in the entire populations (10,202 particles for INO80-Cies6, 10,482 particles for SWR-Cswc2; seeSupplementary Figs 7b and 8bfor all averages). Side length of individual panels is 62.6 nm. (b) Nucleosome-stimulated ATPase activity of the INO80-Cies6subcomplex. (c) DNA-stimulated ATPase activity of the INO80-Cies6subcomplex. Each error bar represents the standard deviation from three independent experiments. WT, wild type. Figure 5: Structural and functional analysis of INO80-C ies6 and SWR-C swc2 subcomplexes. ( a ) Selected class averages of negatively stained INO80-C ies6 and SWR-C swc2 subcomplexes showing extended (upper panels) and compact conformations (lower panels). The numbers are percentages of each conformation in the entire populations (10,202 particles for INO80-C ies6 , 10,482 particles for SWR-C swc2 ; see Supplementary Figs 7b and 8b for all averages). Side length of individual panels is 62.6 nm. ( b ) Nucleosome-stimulated ATPase activity of the INO80-C ies6 subcomplex. ( c ) DNA-stimulated ATPase activity of the INO80-C ies6 subcomplex. Each error bar represents the standard deviation from three independent experiments. WT, wild type. Full size image The Ies6/Arp5 and Swc2/Swc3/Swc6/Arp6 modules both contribute to remodelling activity. As shown previously, a SWR-C complex that lacks the Swc2 module has altered substrate specificity for ATPase activity, and this subcomplex catalyses H2A.Z eviction rather than H2A.Z deposition [24] . In contrast, removal of the Ies6/Arp5 module crippled many of the activities of INO80-C ( Fig. 5b,c and Fig. 6 ). The INO80-C ies6 had a low level of ATPase activity in the absence of nucleic acid, and only minor stimulation of this activity by either DNA or nucleosomes was apparent over a wide range of substrate concentrations ( Fig. 5b,c ). Gel-shift analyses indicated that the INO80-C ies6 subcomplex had only a small defect in binding to nucleosomes ( Fig. 6a ), consistent with a defect in k cat rather than K m ( Table 1 ). Furthermore, the INO80-C ies6 subcomplex was inactive in mononucleosome sliding, nucleosomal array remodelling and dimer exchange assays ( Fig. 6b,c ). These data suggest that the Ies6/Arp5 module is essential for the activity of INO80-C. 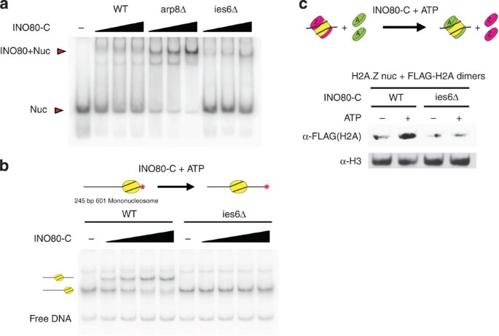Figure 6: The INO80-Cies6subcomplex is inactive in remodelling assays. (a) Nucleosome-binding activity of INO80-C and the INO80-Carp8and INO80-Cies6subcomplexes was analysed by a gel-shift assay. 2 nM 154-bp mononucleosomes were incubated with each complex and subjected to 4% Native-PAGE. (b) Mononucleosome-sliding activity of the INO80-Carp8subcomplex. The assays were performed as described inFig. 3e. (c) Dimer-exchange activity of the INO80-Cies6subcomplex. 5 nM INO80-C wild type (WT) and INO80-Cies6were incubated with 100 nM H2A.Z containing mononucleosomes and 50 nM FLAG-tagged H2A/H2B dimers for 60 min in the presence or absence of 2 mM ATP. Figure 6: The INO80-C ies6 subcomplex is inactive in remodelling assays. ( a ) Nucleosome-binding activity of INO80-C and the INO80-C arp8 and INO80-C ies6 subcomplexes was analysed by a gel-shift assay. 2 nM 154-bp mononucleosomes were incubated with each complex and subjected to 4% Native-PAGE. ( b ) Mononucleosome-sliding activity of the INO80-C arp8 subcomplex. The assays were performed as described in Fig. 3e . ( c ) Dimer-exchange activity of the INO80-C ies6 subcomplex. 5 nM INO80-C wild type (WT) and INO80-C ies6 were incubated with 100 nM H2A.Z containing mononucleosomes and 50 nM FLAG-tagged H2A/H2B dimers for 60 min in the presence or absence of 2 mM ATP. Full size image INO80-C and SWR-C lack helicase activity Biochemical studies have shown that Rvb1 and Rvb2 have the potential to form single or double hexameric rings, and a double hexameric ring of Rvb1/Rvb2 has helicase activity in vitro [25] . An early study reported that INO80-C also has helicase activity [27] , and these authors proposed that this activity might be due to the Rvb1/Rvb2 subunits. A subsequent analysis showed that the ATPase activity of Rvb1 is not required for INO80-C remodelling activity in vitro [12] , indicating that this putative helicase activity was not key for chromatin remodelling. We attempted to address the role of the INO80-C and SWR-C subunit modules in the putative helicase activity of INO80-C. However, using the identical substrates that were previously described [27] , we were unable to detect helicase activity within three independent preparations of either INO80-C or SWR-C ( Fig. 7 ). As a positive control, the human BLM helicase showed robust activity in these assays. We conclude that INO80-C and SWR-C, similar to all other remodelling enzymes, lack helicase activity. 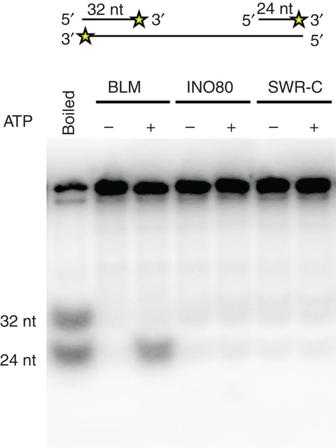Figure 7: INO80-C and SWR-C lack helicase activity. Upper panel shows a schematic diagram of substrates used for the DNA helicase assay. Radiolabelled 32-mer and 24-mer oligonucleotides were annealed to linear, single-stranded ΦX174 DNA. The star denotes the location of the32P label. Native-PAGE (lower panel) showed that both INO80-C and SWR-C were not able to displace any oligonuleotides, whereas human BLM helicase displaced only the 24-mer oligonucleotide showing a 3′ to 5′ helicase activity. Figure 7: INO80-C and SWR-C lack helicase activity. Upper panel shows a schematic diagram of substrates used for the DNA helicase assay. Radiolabelled 32-mer and 24-mer oligonucleotides were annealed to linear, single-stranded ΦX174 DNA. The star denotes the location of the 32 P label. Native-PAGE (lower panel) showed that both INO80-C and SWR-C were not able to displace any oligonuleotides, whereas human BLM helicase displaced only the 24-mer oligonucleotide showing a 3′ to 5′ helicase activity. Full size image Our studies have shown that the INO80-C and SWR-C remodelling enzymes share striking similarities in both their overall dimensions and subunit architecture. Both enzymes exist as a heterogeneous population of elongated and compact forms, and each contains a single ring of AAA + ATPase subunits as a dominant structural feature. Notably, the overall architectures of INO80-C and SWR-C, although similar to each other, are quite distinct from that of the SWI/SNF family of enzymes, reinforcing the view that each family of chromatin remodelling enzymes harbours distinct structural features that may be key for their specific activities and/or regulation. Two recent studies have also described structural features of the yeast INO80-C and SWR-C remodelling enzymes [11] , [23] . EM analysis of SWR-C by the Leschziner group shows several similarities to our analysis [22] . They find that SWR-C is highly heterogeneous, and they circumvented this issue by employing a formaldehyde gradient method to fractionate SWR-C, and fractions that appeared more homogeneous by EM were selected for analysis. This method resulted in a population of SWR-C that was compact, and it appears to have eliminated the more heterogeneous population of extended molecules. Similar to our analysis, SWR-C was reported to contain a single heterohexameric Rvb1/Rvb2 ring. Similar to our study, the Hopfner group reported that INO80-C exists as both elongated and compact (bent) forms, and the prominent ‘head’ group is composed of the Rvb1 and Rvb2 subunits [11] . In addition, they find that the Arp8/Arp4/Act1 module is localized to the extended tail domain, and that the Ies6/Arp5 module maps to the base of the head domain, as predicted from previous biochemical studies [10] . Based primarily on the size of the head, and in contrast to our study, these authors proposed that the Rvb1/Rvb2 head group is composed of a double heterohexameric ring. The authors do note, however, that an Rvb1/Rvb2 dodecamer would have to be compacted or locked in a particular conformation in order to fit into the volume they assigned in their map to the INO80-C head. Interestingly, the side view of the Rvb1/Rvb2 head within our INO80-C average appears to show two stacks of symmetrical density ( Fig. 2a ). However, by mass spectrometry, we detect a stoichiometry for Rvb1/Rvb2 that, although higher than would be expected for a single ring, is much less than expected for a dodecamer. This may reflect additional molecules of Rvb1/Rvb2 that might interact with the heterohexamer ring. One possibility is that the second ‘ring’ of density seen in the INO80-C average may not represent a second hexamer but may be due to the AAA + insertion domains that are contributed by each Rvb monomer. This notion is supported by EM images of the human RuvBL dodecamer that show three distinct layers of density, where the two heterohexameric rings flank a central region composed of the insertion domains [28] . Although the insertion domains of RuvBL and Rvb1/Rvb2 are similar in size, this tripartite view is not observed in our averages of INO80-C or SWR-C. Importantly, the presence of single Rvb1/Rvb2 rings within both INO80-C and SWR-C is most consistent with their similar biochemical activities, similar subunit structure and the sequence relatedness of the Ino80 and Swr1 ATPase subunits that form binding platforms for the Rvb1/Rvb2 ring. Early studies of an INO80-C complex that lacks the Arp8/Arp4/Act1 module indicated that Arp8 was essential for the ATPase and remodelling activities of INO80 (ref. 10 ). Consequently, a large number of genetic studies have employed arp8Δ strains in order to dissect the role of INO80-C in gene transcription or genome stability pathways. However, our quantitative ATPase and remodelling assays have revealed that the absence of the Arp8/Arp4/Act1 module reduces, but does not eliminate, the ATPase and remodelling activities of INO80-C. We found that the Arp8/Arp4/Act1 module enhances the K m of INO80-C for nucleosomes and DNA, but INO80-C that lacks the Arp8/Arp4/Act1 module exhibits 13–50% remodelling activity in a variety of quantitative assays. Notably, a recent, independent study also confirms that the Arp8/Arp4/Act1 module is not essential for ATPase and remodelling activity [11] . Our biochemical data are also consistent with the differing genetic phenotypes of ino80Δ and arp8Δ mutants. For instance, whereas an ino80Δ appears to be lethal in many strain backgrounds, an arp8Δ is viable and has only a moderate growth defect. Likewise, in strain backgrounds in which an ino80Δ is viable, an arp8Δ assayed in parallel shows less severe growth sensitivity to a variety of genotoxic agents [4] , [29] , [30] . Indeed, Ino80 is recruited to a DNA double-strand break in the absence of Arp8, suggesting that Arp8 is also not required for recruitment to sites of DNA damage [29] . In contrast, an ies6Δ mutant has phenotypes that appear to be identical to that of an ino80Δ mutant, consistent with our finding that the Ies6/Arp5 module is essential for the ATPase and remodelling activities of INO80-C [30] . The Ies6 and Swc2 subunits share homology with the metazoan YL1 protein that is a subunit of the mammalian Tip60/p400 histone acetyltransferase/chromatin remodelling enzyme and the SRCAP chromatin remodelling enzyme [9] . This homology is also shared by the mammalian homologue of Ies6 that is found within human INO80-C [31] . The Ies6 and Swc2 subunits have been reported to bind histones and DNA, with Swc2 showing a preference for binding H2A.Z compared with H2A [9] . Such binding specificity is consistent with our recent study showing that Swc2 prevents H2A.Z eviction following SWR-C-mediated deposition [24] . We found here that Ies6 promotes both the DNA- and nucleosome-stimulated ATPase activity of INO80-C, and that this subunit is essential for chromatin-remodelling activities. Consistent with a previous study, our data also show that the Ies6 module plays only a minor role in the nucleosome-binding activity of INO80-C, as assayed by gel-shift assays [11] . In contrast, a recent study reported that human Ies6 appears to play a more dominant role in nucleosome recognition compared with the yeast homologue [33] , but like the yeast homologue, it is key for hINO80 remodelling activity. This differing role for yeast and human Ies6 may reflect the fact that the nonconserved, yeast Nhp10 subunit, dispensable for INO80-C remodelling activity in vitro , appears to dominate the nucleosome-binding activity of INO80-C assayed by gel shift [10] , [11] . Our structural studies indicate that Ies6 influences large-scale conformational changes within INO80-C, promoting formation of an extended form. Loss of the related Swc2 subunit from SWR-C also appears to lead to an increased prevalence for compact forms, although the magnitude of the effect is less dramatic. Based on a recent model for nucleosome recognition by INO80-C [11] , these data suggest a model in which Ies6 and Swc2 help to maintain an active, extended form of the enzyme that is competent for functional interactions with a nucleosomal substrate ( Fig. 8 ). In this model, the compact conformations that are observed in the absence of nucleosomes may represent an inactive conformation, and the YL1-related subunits, Ies6 and Swc2, function as a ‘hinge’ that responds to nucleosome binding, catalysing productive interactions with the catalytic ATPase domain. Such a conformational change, involving subunit modules that contain Actin-related proteins (Arps), is reminiscent of the coupling role proposed for the Arp7/Arp9 module of the yeast SWI/SNF and RSC remodelling enzymes [8] . 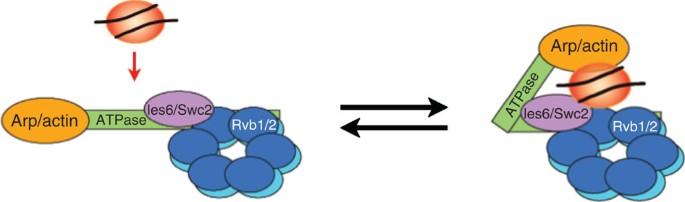Figure 8: Model depicting the proposed conformational change of INO80-C that is coupled to nucleosome binding. The model proposes that the Ies6/Arp5 module helps to maintain an active, extended form that is competent for functional interactions with a nucleosome. This module is postulated to function as a ‘hinge’ that responds to nucleosome binding, catalysing productive interactions with the catalytic ATPase domain. Figure 8: Model depicting the proposed conformational change of INO80-C that is coupled to nucleosome binding. The model proposes that the Ies6/Arp5 module helps to maintain an active, extended form that is competent for functional interactions with a nucleosome. This module is postulated to function as a ‘hinge’ that responds to nucleosome binding, catalysing productive interactions with the catalytic ATPase domain. Full size image Protein purifications INO80-C and SWR-C were purified from yeast strains encoding TAP-tagged Ino80 and TAP-tagged Swr1 (Open Biosystems), respectively [34] . Cultures were grown in Yeast Extract/Peptone/Dextrose (YPD) media, and harvested cells were lysed in buffer E (20 mM HEPES, pH 7.5, 350 mM NaCl, 10% glycerol, 0.1% Tween and 1 mM dithiothreitol (DTT)) and protease inhibitors by grinding in the presence of liquid nitrogen. Lysates were clarified at 40,000 g at 4 °C for 1 h. Cleared lysates were incubated with IgG-Sepharose (GE Healthcare) and eluted by TEV protease cleavage. The elutions were incubated with calmodulin affinity resin (Stratagene) in buffer E plus 2 mM CaCl 2 and eluted in buffer E plus 10 mM EGTA. Samples were dialysed against buffer E. Subunit compositions were confirmed by SDS–PAGE and mass spectrometry. Recombinant yeast and Xenopus histones were expressed in BL21 Escherichia coli cells [35] , [36] , [37] . Expressed histones were purified as inclusion bodies, solubilized in unfolding buffer (7 M guanidinium hydrochloride, 20 mM Tris-HCl, pH 7.5, 10 mM DTT), and dialysed against urea dialysis buffer (7 M urea, 10 mM Tris-HCl, pH 8.0, 0.1 M NaCl, 1 mM EDTA, 0.2 mM phenylmethylsulphonyl fluoride and 5 mM 2-mercaptoethanol). Samples were injected into tandemly connected Q Sepharose and SP Sepharose columns, and eluted from SP Sepharose by a linear salt gradient. Histone fractions were dialysed against water plus 0.2 mM phenylmethylsulphonyl fluoride and 5 mM 2-mercaptoethanol, and lyophilized. The four histones were mixed in equimolar ratios in unfolding buffer, dialysed against refolding buffer (2 M NaCl, 10 mM Tris-HCl, pH 7.5, 1 mM EDTA and 5 mM 2-mercaptoethanol) and purified through a Superdex-200 column. Nucleosomes were reconstituted by mixing octamers with DNA in 1:1 ratio in Hi buffer (2 M NaCl, 10 mM Tris-HCl, pH 7.5, 1 mM EDTA, 0.05% NP-40 and 5 mM 2-mercaptoethanol) and 0.5 mg ml −1 BSA, and dialysing against a liner salt gradient buffer from Hi buffer to Lo buffer (50 mM NaCl, 10 mM Tris-HCl, pH 7.5, 1 mM EDTA, 0.05% NP-40 and 5 mM 2-mercaptoethanol) for 20 h. ATPase assays ATPase assays were performed as previously described [38] . Mononucleosomes were reconstituted by salt dialysis onto a 154-bp DNA fragment containing the 601 nucleosome-positioning sequence. DNA (154 bp 601 template) or mononucleosomes were incubated with remodelling enzymes in buffer A (10 mM Tris-HCl, pH 8.0, 70 mM NaCl, 5 mM MgCl 2 , 0.1 mg ml −1 BSA and 1 mM DTT) at 30 °C. ATP-hydrolysis rates were determined over three linear time points. Nucleosome-remodelling assays Nucleosome-sliding assays were performed as previously described [39] . Briefly, mononucleosomes were reconstituted onto a 245-bp 32 P-labelled DNA fragment containing the 601 nucleosome-positioning sequence at the fragment end. Mononuleosomes (1 nM) were incubated with remodelling enzymes and 2 mM ATP in buffer A for 15 min at 30 °C. The reactions were quenched with 5% glycerol and 1 mg ml −1 salmon sperm DNA, incubated for 5 min at 30 °C, and resolved on 5% Native-PAGE in 0.5 × tris-borate-EDTA (TBE). Sal I restriction enzyme accessibility assays were performed as described [26] . Nucleosomal arrays were reconstituted by salt dialysis onto 32 P-labelled 208-11 templates. Nucleosomal arrays (5 or 50 nM) were incubated in buffer A with 5 nM remodelling enzymes, 20 KU ml −1 of Sal I and 2 mM ATP at 30 °C. At each time point, the reactions were stopped by the addition of phenol. The extracted DNA was resolved on 1% agarose gels. Gels were dried and exposed to film. The percentage of digested DNA was quantified by phosphorimager analysis. Gel-shift assays for nucleosome binding 32 P-labelled mononucleosomes (154 bp DNA) were incubated with remodelling enzymes in buffer A for 15 min at room temperature. The reactions were resolved on 4% Native-PAGE in 0.5 × TBE. Gels were dried and exposed to film. In vitro dimer-exchange assays The dimer-exchange assay was performed as previously described [4] . H2A.Z-containing mononucleosomes (200 bp DNA, 100 nM) were incubated with remodelling enzymes, free FLAG-tagged H2A/H2B dimers (50 nM) and 2 mM ATP in buffer A at 30 °C. The reactions were subjected to 5% Native-PAGE in 0.5 × TBE. The gels were soaked in SDS buffer (25 mM Tris, pH 8.8, 192 mM glycine, 0.1% SDS), and then transferred onto polyvinylidene difluoride membranes for western blotting. Western blotting was performed using a commercially available antibody raised against the FLAG epitope (Sigma, Cat#3165) or yeast histone H3 (AbCam, Cat# ab1791). Electron microscopy All samples were mildly cross-linked for EM analysis. Complexes were cross-linked by adding a final concentration of 0.04% glutaraldehyde (Electron Microscopy Sciences) directly into the purified protein fraction immediately after the final column elution, followed by incubation on ice. After 10 min, Tris-HCl, pH 8.0, was added to a final concentration of 50 mM to stop the reaction. For negative staining, samples were adsorbed to glow-discharged carbon-coated copper grids and stained with 0.75% (w/v) uranyl formate solution as described [40] . All images were collected with a Tecnai T12 electron microscope (FEI) operated at an acceleration voltage of 120 kV. For 2D analysis of INO80-C, SWR-C and the INO80-C arp8 subcomplex, images were recorded on imaging plates at a nominal magnification of × 67,000 and a defocus of about —1.5 μm using low-dose procedures. Imaging plates were read out with a scanner (DITABIS) using a step size of 15 μm, a gain setting of 20,000 and a laser power setting of 30% (ref. 41 ). The images were binned over 2 × 2 pixels, yielding a pixel size of 4.5 Å at the specimen level. For 2D analysis of the INO80-C ies6 and the SWR-C swc2 subcomplexes, images were collected with a 4 K × 4 K charge-coupled device (CCD) camera (Gatan) at a nominal magnification of × 42,000 ( × 57,555 after calibration) and a defocus of about −1.5 μm using low-dose procedures. The pixel size at the specimen level was 2.61 Å. For 3D reconstructions, 217 60°/0° image pairs for the INO80-C complex and 256 pairs for the SWR-C complex were collected on CCD camera at a nominal magnification of × 30,000 ( × 40,607 after calibration) and a defocus of about 1.5 μm using low-dose procedures. Image processing For 2D analysis, interactive particle picking was performed using BOXER, the display programme associated with the EMAN software package [42] . For INO80-C, 10,128 particles were selected, and 9,370 particles were selected for the INO80-C arp 8 subcomplex. For SWR-C, 20,412 particles were selected. For all three data sets, particles were windowed into 128 × 128-pixel images, which were normalized, rotationally and translationally aligned, and subjected to ten cycles of multi-reference alignment using the SPIDER software package [43] . Each round of multi-reference alignment was followed by K-means classification specifying 100 output classes. The references used for the first multi-reference alignment were randomly chosen from the particle images. For the INO80-C ies6 subcomplex, 10,202 particles were selected, and 10,482 particles were selected for the SWR-C swc2 subcomplex, both from 4 K × 4 K CCD images. For these two data sets, particles were windowed into 240 × 240-pixel images. The particles were then subjected to the same alignment and classification procedure described above. In both cases, 100 output classes were specified. To increase the definition of structural features of the head domain of INO80-C and SWR-C, classes showing averages with well-defined head domains were selected from each data set, and the particles belonging to these classes were combined, 5,254 for INO80-C and 5,621 for SWR-C, and subjected to further image analysis. The particle images were centred on their head domain, and then rotationally and translationally aligned as described above, using a circular mask to exclude from this analysis parts of the particles other than the head domain. Each round of multi-reference alignment was followed by K-means classification as described above, specifying 25 output classes for INO80-C and 20 classes for SWR-C. Some of the resulting class averages showed the Rvb1/Rvb2-ring in the top view with a clear sixfold symmetry and some showed the side view, revealing two stacked rings. Two class averages from each data set were selected for Fig. 2a,b . To estimate the percentage of particles in different conformations in each data set, only particles belonging to classes with well-resolved features ( Supplementary Figs 2–5 ) were assigned to represent either ‘extended’ or ‘compact’ conformations. The percentages are given with respect to the total particle numbers, which include particles that could not unambiguously be assigned to one of the two conformations. For 3D reconstruction, 9,384 particle pairs for INO80-C complex and 24,052 particle pairs for the SWR-C complex were interactively selected using WEB [43] . Particles were then windowed into 160 × 160-pixel images. One hundred output classes were specified for INO80-C and 150 output classes for SWR-C. In all, 8 out of the 100 classes from the INO80-C data set and 3 out of the 150 classes from the SWR-C data set looked similar, and particles in these classes were combined (796 particles for INO80-C and 250 particles for SWR-C) for 3D reconstruction of each complex. The 3D reconstructions were calculated with the particles selected from the images of the tilted specimen using the backprojection and angular refinement procedures in SPIDER. The resolution of the INO80-C density map was 33 Å and that of the SWR-C density map was 36 Å according to the Fourier shell correlation=0.5 criterion [44] . The final maps shown were low-pass filtered to their respective resolutions. Mass spectrometry analyses Three independent samples of INO80-C and SWR-C were purified from TAP-tagged strains as described above, but the final samples were treated with 0.1 U Benzonase (Sigma, Cat#E8263) at 37 °C for 30 min followed by trichloroacetic acid (Sigma, Cat#T0699) precipitation and stored overnight at 4 °C. The next day, trichloroacetic acid was removed by centrifugation and samples were washed twice with ice-cold acetone, air-dried and resuspended in 100 mM Tris-HCl, pH 8.5, and 8 M urea. To reduce and alkylate sulfhydryl bonds, samples were incubated for 30 min first with 5 mM tris-(2-carboxyethyl)-phosphine hydrochloride (Pierce, Cat#20490) and then with 10 mM chloroacetamide (Sigma, Cat#C0267) at room temperature in the dark. Protein samples were then digested using sequencing grade Endoproteinase Lys-C (Roche, Cat#11047817001) (0.5 μg) for 6 h at 37 °C, diluted with 100 mM Tris, pH 8.5, to reduce the concentration of urea to 2 M, supplemented with 2 mM CaCl 2 and incubated overnight with sequencing grade Trypsin protease (Promega Cat#V5111; 0.5 μg) at 37 °C. Reactions were quenched by adding formic acid (J.T.Baker, Cat#0129-01) to a final concentration of 5% (v/v). Samples were pressure-loaded on triple-phase 100 μm fused silica microcapillary columns and placed in-line with an LTQ Velos-Orbitrap Elite hybrid mass spectrometer equipped with a nano-liquid chromatography electrospray ionization source (Thermo Scientific) that was coupled with a quaternary Agilent 1,260 infinity series HPLC. Multidimensional protein identification technology analyses were performed using an 11-step chromatography (including a final wash step) run as described [45] . An Orbitrap-elite instrument at 60,000 resolution was used to record full MS spectra on peptides over a range of 400–1,600 m / z followed by collision-induced dissociation fragmentation on the 1st to 10th most intense ions (35% collision energy in the ion trap) that were selected from the full MS scan with Dynamic exclusion enabled for 90 s (ref. 46 ). The RAW files from the run were extracted into .ms2 file format using in-house developed software called RawDistiller [47] . SEQUEST algorithm (version 27 (ref. 48 )) was used to search and interpret the MS/MS spectra with a peptide mass tolerance of 10 p.p.m. and ±0.5 a.m.u. for fragment ions without imposing any enzyme specificity. During searching, static modification (+57.02146 Da for carboxamidomethylation of cysteine) and dynamic modification (+15.9949 Da for oxidized methionine) were employed. The database used for the search was from the National Center for Biotechnology Information (release date 26 April 2011) and contained a total of 11,990 sequences, out of which 5,819 were nonredudant Saccharomyces cerevisiae protein sequences. The rest of the sequences comprised of 176 commonly found contaminants (IgGs, human keratin, proteolytic enzymes and so on), shuffled sequences of S. cerevisiae proteins and contaminants to estimate false discovery rates. Peptide/spectra matches and label-free quantification using the spectral counting method were performed as described [49] . All the RAW and .ms2 files have been uploaded in the MassIVE database and can be found using the following reference numbers: INO80-C submission, MSV000079018; Swr-C submission, MSV000079019. Files are password protected until publication. How to cite this article: Watanabe, S. et al . Structural analyses of the chromatin remodelling enzymes INO80-C and SWR-C. Nat. Commun. 6:7108 doi: 10.1038/ncomms8108 (2015).